Elucidating tumor heterogeneity from spatially resolved transcriptomics data by multi-view graph collaborative learning Spatially resolved transcriptomics (SRT) technology enables us to gain novel insights into tissue architecture and cell development, especially in tumors. However, lacking computational exploitation of biological contexts and multi-view features severely hinders the elucidation of tissue heterogeneity. Here, we propose stMVC, a multi-view graph collaborative-learning model that integrates histology, gene expression, spatial location, and biological contexts in analyzing SRT data by attention. Specifically, stMVC adopting semi-supervised graph attention autoencoder separately learns view-specific representations of histological-similarity-graph or spatial-location-graph, and then simultaneously integrates two-view graphs for robust representations through attention under semi-supervision of biological contexts. stMVC outperforms other tools in detecting tissue structure, inferring trajectory relationships, and denoising on benchmark slices of human cortex. Particularly, stMVC identifies disease-related cell-states and their transition cell-states in breast cancer study, which are further validated by the functional and survival analysis of independent clinical data. Those results demonstrate clinical and prognostic applications from SRT data. The recent technological innovation of SRT platform, including sequencing-based technology (e.g., 10X Genomics Visium and Stereo-seq) and imaging-based technology (e.g., STARmap) [1] , [2] , [3] allows profiling gene expression patterns in the spatial contexts of tissue [4] . These resulting multiple types of profiles: histology, spatial location, and gene expression, provide novel insights into the organization of cells and developmental biology, especially for the evolution of the tumor [5] , [6] , [7] . However, SRT data analysis for biology discovery remains challenging due to its low throughput, little sensitive, much sparse, and noisy [8] , [9] . Recently, several computational methods have been designed to analyze SRT data [8] . For example, Giotto uses a similar processing strategy to single-cell RNA-seq (scRNA-seq), for feature selection, dimension reduction, and unsupervised clustering [10] . BayesSpace utilizes a fully Bayesian statistical method to enhance the spatial measurement via spatial neighborhood structure for clustering analysis [9] . SpaGCN adopting a graph convolutional network (GCN) approach integrates gene expression, spatial location, and histology to identify spatial domains and spatially variable genes (SVGs) [11] . stLearn integrates features of histology with spatial location to normalize gene expression data, and followed by clustering [12] . Squidpy brings together omics and image analysis tools to enable scalable description of spatial transcriptomics and proteomics data [13] . ClusterMap incorporates physical location and gene identity of RNAs to identify biologically meaningful structures from image-based in situ transcriptomics data [14] . DR-SC [15] and SC-MEB [16] utilizing latent hidden Markov random field model integrates gene expression and spatial location for spatial clustering. STAGATE [17] combines gene expression and spatial information to detect spatial domains via graph attention auto-encoder framework. While these methods have many interesting findings, the lack of visual features that can be effectively and globally extracted from histology, efficient multi-view information fusion, and the biological contexts such as global positional information within a tissue, limits their disentangling capabilities in developmental biology. On the other hand, GCN-based models have appeared as powerful tools to learn the representations of scRNA-seq data (i.e., by scGNN) [18] and SRT data (i.e., by SpaGCN) [11] , however, these methods usually study networks with a single type of proximity between nodes, namely single-view network. Although SpaGCN proposes an RGB color space averaging strategy to convert histological data into the same measurement space as 2D space in the tissue slice as a third dimension before calculating the similarity between any two spots, to a certain extent, this strategy discards the texture features in each spot, i.e., the strategy extracts the color features from color space without fully utilizing the spatial distribution of gray tone variations within a specified area namely texture features [19] . Besides, in SRT studies, \(K\) -nearest spots that are physically closest to the central spot are not necessarily the same as those that are the most histologically similar to the spot, and the distance evaluation metrics between multi-view data are also not the same, thus yielding networks with multiple views. Moreover, the contributions of neighboring spots to determine the cell type to which the central spot belongs are not identical, which is consistent with the assumption of graph attention network (GAT) [20] , [21] . More importantly, the quality of the information in different views may be different, hence, it would be preferable that one novel model can learn the representations for each view by GAT, and meanwhile collaboratively integrate multiple networks to learn robust representations by automatically training the weights of different views [22] . We reason that (i) cells belonging to the same cell type but distributed in different areas and interacting with different cell types in the tissue may have different cell-states [8] ; (ii) the determination of each cell type (or cell-state) to which each cell belongs, is related to its size, shape, and arrangement (i.e., tightness or looseness), hence the texture data of histology has rich information to characterize cell type or cell-state [23] ; and (iii) the colors of the antibodies on the immunofluorescence staining of the tumor sample can roughly mark the tumor position in the tissue, yielding region segmentation indicating biological contexts related to the tumor development. In this work, we introduce stMVC ( S patial T ranscriptomics data analysis by M ultiple V iew C ollaborative-learning), a framework that integrates four-layer information to elucidate tissue heterogeneity by attention-based multi-view graph collaborative learning, i.e., histology, gene expression data, spatial location, and region segmentation (e.g., tumor position) indicating biological contexts. The features of stMVC are as follows: (i) for each spot, globally learning efficient visual features while removing artifacts from histology by data augmentations and contrastive learning; (ii) learning robust representations for each spot by training the weights of multi-view graphs including histological-similarity-graph (HSG) by visual features and spatial-location-graph (SLG) by physical coordinates, via attention-based collaborative learning strategy, under semi-supervision of region segmentation; (iii) for samples of human ovarian endometrial adenocarcinoma (OEAD) and breast invasive ductal carcinoma (IDC), identifying cancer-related cell-states (i.e., stemness, migration, and metastasis) missed by competing methods, and also transition cell-states, which are further validated by clinical data from other independent studies, demonstrating potential clinical and prognostic applications from SRT data; and (iv) for sample of mouse primary visual cortex, enabling us to detect layer-specific inhibitory neurons. In particular, such a multi-view graph collaborative learning method is a flexible framework that is able to integrate not only SRT data from multi-sources or spatial multi-omics data but also spatial epigenomics or proteomics data. Overview of stMVC model stMVC collaboratively integrates histological image ( \(I\) ), spatial locations ( \(S\) ), and gene expression data ( \(X\) ), through the semi-supervision learning from biological contexts (i.e., region segmentation, \(Y\) , see Manual region segmentation) within a tissue, to clarify tissue heterogeneity (Fig. 1a–d ). Specifically, we (1) learned the visual features ( \({h}_{i}\) ) for each spot image ( \({i}_{i}\) ) by ResNet-50 model [24] (an efficient computer vision framework) that was trained by maximizing the agreement between differently augmented views of the same histological spot image, and then constructed HSG based on \({h}_{i}\) (Fig. 1b ); and (2) captured the spot proximities encoded in either histology or spatial location, as well as the low-dimensional features ( \({z}_{i}\) ) from gene expression data by autoencoder (AE) (see Supplementary Methods ), and then simultaneously integrated these two graphs for the robust representations ( \({r}_{i}\) ) by automatically learning the weight of view-specific representations ( \({{p}_{i}}^{1}\) and \({{p}_{i}}^{2}\) ) from two graphs via attention, under semi-supervision of region segmentation (Fig. 1c ). Hence, \(R\) is a low-dimensional feature representing the variation of these four-layer profiles, which is used to represent each spot as a point in the low-dimensional space, for spatial clustering and visualization, where each cluster is considered as a spatial domain. Subsequently, for each spot, we denoised gene expression data by its 15 nearest neighboring spots that are calculated based on the distance of robust representations, and then identified SVGs that are over-expressed in a domain by differential expression analysis (Fig. 1d ). Fig. 1: Overview of stMVC model. a Given each SRT data with four-layer profiles: histological images ( \(I\) ), spatial locations ( \(S\) ), gene expression ( \(X\) ), and manual region segmentation ( \(Y\) ) as the input, stMVC integrates them to disentangle tissue heterogeneity, particularly for the tumor. b stMVC adopts SimCLR model with feature extraction framework from ResNet-50 to efficiently learn visual features ( \({h}_{i}\) ) for each spot ( \({v}_{i}\) ) by maximizing agreement between differently augmented views of the same spot image ( \({i}_{i}\) ) via a contrastive loss in the latent space ( \({l}_{i}\) ), and then constructs HSG by the learned visual features \({h}_{i}\) . c stMVC model adopting SGATE model learns view-specific representations ( \({{p}_{i}}^{1}\) and \({{p}_{i}}^{2}\) ) for each of two graphs including HSG and SLG, as well as the latent feature from gene expression data by the autoencoder-based framework as a feature matrix, where a SGATE for each view is trained under weak supervision of the region segmentation to capture its efficient low-dimensional manifold structure, and simultaneously integrates two-view graphs for robust representations ( \({r}_{i}\) ) by learning weights of different views via attention mechanism. d Robust representations \(R\) can be used for elucidating tumor heterogeneity: detecting spatial domains, visualizing the relationship distance between different domains, and further denoising data. Full size image To emphasize the advantages of stMVC, we designed several comparative methods in our experiments: (i) the mean of all view-specific representations was used as a comparison to assess the efficiency of the attention-based multi-view integration strategy enabling the network to focus on the key features for characterizing tissue structure, which is named stMVC-M; (ii) the single-view graph representations by semi-supervised graph attention autoencoder (SGATE) for either SLG (SGATE-SLG) or HSG (SGATE-HSG) were utilized to assess the effectiveness of the robust representations by multi-view graphs; (iii) the naïve HSG (SGATE-HSG-N) constructed based on the visual features by the ResNet-50 model (pre-trained by ImageNet [25] ) was used to evaluate the quality of the visual features by our ResNet-50 model trained by histological images; and (iv) the low-dimensional representations encoded from gene expression data, via AE or semi-AE extended from AE through adding a classifier on bottleneck layer (see Supplementary Methods ), were used to check if or not the components of semi-supervised learning and graph attention mechanism used by SGATE-SLG are responsible for capturing complex structure of SRT data. stMVC reveals the trajectory relationship between different spatial domains The most important feature of the stMVC model is that the learned low-dimensional representations can reveal the trajectory relationship between different spatial domains through semi-supervised biological contexts. To assess the performance of stMVC, we applied it to process 12 slices of the human dorsolateral prefrontal cortex (DLPFC) dataset, each of which was manually annotated with six layers and white matter (WM), and the spatial adjacency and chronological order among these layers are WM → Layer6 → Layer5 → Layer4 → Layer3 → Layer2 → Layer1 (Fig. 2a ) [26] , [27] . By default, through the semi-supervised learning of 70% of the annotation (Supplementary Fig. 1 , Evaluation of proportion of labels for model training in Supplementary Note 1 ), stMVC, stMVC-M, and the three SGATE-based single-view models extracted 10-dimensional features from the input. For comparison, we also applied six recently developed methods including BayesSpace, Giotto, stLearn, Squidpy, DR-SC, and STAGATE for spatial clustering or visualization with the default parameters. Subsequently, we predicted cell clusters by the Louvain algorithm, evaluated clustering accuracy including ROGUE [28] and average silhouette width (ASW) [29] by calculating the similarity of the transcriptome and multi-view joint features between spots within each predicted cell cluster, respectively, and then visualized these low-dimensional features by mapping them into two uniform manifold approximation and projection (UMAP) spaces. Fig. 2: stMVC is able to detect spatial domains, visualize the relationship distance between different domains, and denoise data on the DLPFC dataset. a Annotation of seven DLPFC layers in slice 151673 by the previous study [26] , and the spatial adjacency and chronological order between these layers are WM → Layer6 → Layer5 → Layer4 → Layer3 → Layer2 → Layer1. b Boxplot of clustering accuracy in terms of average silhouette width (ASW) for assessing the closeness of multi-view joint features of same cluster compared to the other clusters, on all n = 12 samples. In the boxplot, the center line, box limits and whiskers separately indicate the median, upper and lower quartiles and 1.5 × interquartile range. c Spatial domains detected by BayesSpace, Giotto, stLearn, Squidpy, DR-SC, STAGATE, AE, semi-AE, the three SGATE-based single-view models, stMVC-M, and stMVC on slice 151673. d Scatter plot of the two-dimensional UMAP extracted from the latent features by Giotto, stLearn, Squidpy, DR-SC, STAGATE, AE, semi-AE, three SGATE-based single-view models, stMVC-M, and stMVC on slice 151673. Note that the trajectory between seven layers or domains is consistent with ( a ), and for each method, the predicted clusters and their colors are the same as ( c ). Note that subplot b – d BayesSpace cannot calculate ASW and visualized using UMAP. e Boxplot of the Gini-index (GI) score of gene expression data denoised by stLearn, BayesSpace, STAGATE, the three SGATE-based single-view models, stMVC-M, and stMVC for n = 12 samples. The higher GI score, the better the denoised data. In the boxplot, the center line, box limits and whiskers indicate the median, upper and lower quartiles and 1.5 × interquartile range, respectively. f Spatial expression of layer-specific genes: [26] PCP4 , PVALB , ENC1 , CCK , KRT17 , and MOBP for slice 151673 data denoised by stMVC, where we also provide raw data as a comparison. Source data are provided as a Source Data file. Full size image In summary (Fig. 2b–d and Supplementary Figs. 2 – 4 ), we found that (i) the clustering accuracy of stMVC is higher than that of the three SGATE-based single-view models, AE, semi-AE, BayesSpace, Giotto, stLearn, Squidpy, DR-SC, and STAGATE, among which ASW for the joint features is the highest while ROGUE for the transcriptomics is similar to other tools, indicating that our multi-view graph collaborative learning model did capture more useful information beyond transcriptomics data than that from single-view graph model; (ii) stMVC performs better than stMVC-M, especially in detecting the precise structure, e.g., Layer4 and Layer6 on slice 151673, demonstrating that the attention-based multi-view integration strategy enables the network to capture critical features for clarifying tissue structure, compared to those by the mean-based strategy; (iii) SGATE-HSG performs better than SGATE-HSG-N, which indicates that our trained visual features extraction model adopted from ResNet-50 by data augmentations and contrastive learning did learn more rich visual features than those from naïve ResNet-50 model pre-trained by ImageNet; (iv) SGATE-SLG performs better than semi-AE and AE, while AE performs worst, indicating that semi-supervised learning and graph attention mechanism are considered responsible for capturing data structure; and (v) each spatial domain is assigned almost by different feature embeddings from stMVC, stMVC-M, and SGATE-SLG model, compared to Giotto, stLearn, Squidpy, DR-SC, STAGATE, AE, semi-AE, and the two HSG-based models, and the distance between different domains of stMVC can reflect the trajectory of chronological order, which shows that stMVC can clarify the complex relationship between different spatial domains. We further assessed the quality of the denoised data from stMVC by our defined Gini-index (GI) scores based on how far the expression distribution of layer-specific genes deviated from a totally equal distribution, where the higher the GI score, the more layer-specific the distribution of gene expression (see Evaluation of denoising of gene expression data). Overall, we observed that stMVC, stMVC-M, and SGATE-SLG have comparable performance, and those three methods perform better than BayesSpace, STAGATE and the two HSG-based models, while stLearn performs worst. For instance, some known layer marker genes such as PCP4 , PVALB , ENC1 , CCK , KRT17 , and MOBP [26] are more specifically expressed in their corresponding spatial location on slice 15,1673, compared with those by BayesSpace and STAGATE (Fig. 2e, f and Supplementary Fig. 5 ). stMVC contributes to detecting cell-states missed by competing methods To illustrate that stMVC is able to clarify cancer cells that are distributed at different positions in the tissue, we further analyzed ovarian cancer (i.e., OEAD) and breast cancer (i.e., IDC) publicly published by 10X Genomics. We separately annotated 18 and 16 regions for ovarian and breast cancer based on our segmentation strategy detailed in Manual region segmentation, where for breast cancer, 15 tumor regions were classified into three different types: invasive carcinoma, carcinoma in situ, and benign hyperplasia by the previous study [9] (Fig. 3a, h and Supplementary Figs. 6a and 8a ). We treated the annotated regions as rough labels, and randomly selected 70% of them to supervise the training of the stMVC. stMVC, stMVC-M, and the three SGATE-based single-view models extracted 18- and 16- dimensional features from ovarian and breast cancer, respectively. Subsequently, we predicted cell clusters by the Louvain algorithm and visualized these low-dimensional features by mapping them into two-dimensional UMAP. For comparison, we also applied Giotto, DR-SC, Squidpy, stLearn, BayesSpace, and STAGATE for spatial clustering or visualization. Fig. 3: stMVC enables the detection of cell-states distributed in different spatial domains on ovarian and breast cancers. a Immunofluorescent staining of the tissue section and 17 manually segmented tumor regions. The intensity of DAPI, cytokeratin, and CD45 is shown in blue, green, and yellow. b Spatial clustering by DR-SC, Squidpy, stLearn, BayesSpace, STAGATE, and stMVC. c UMAP visualization of latent features by stMVC. Each domain is outlined by the region it belongs to, i.e., tumor or non-tumor. d Heatmap of average gene expression of signature genes from 16 domains by stMVC. Rows and columns indicate genes and domains. e UMAP plot of average expression of signature genes for domains 11 and 12 in scRNA-seq data of 4081 epithelial cells from one independent ovarian cancer. f Enrichment of infiltrating stromal and immune cells in each domain compared to the total distribution of those in four domains. The ratio is calculated by chi-square test [85] . The larger the ratio, the more cells are enriched in the domain. 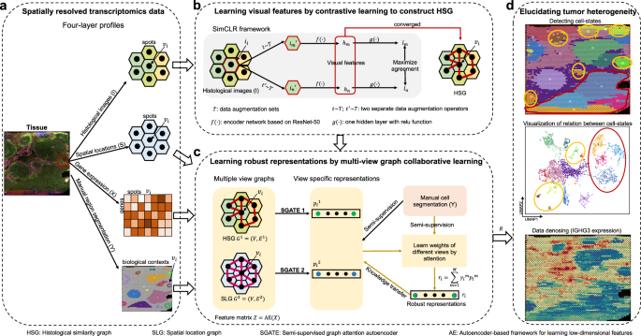Fig. 1: Overview of stMVC model. aGiven each SRT data with four-layer profiles: histological images (\(I\)), spatial locations (\(S\)), gene expression (\(X\)), and manual region segmentation (\(Y\)) as the input, stMVC integrates them to disentangle tissue heterogeneity, particularly for the tumor.bstMVC adopts SimCLR model with feature extraction framework from ResNet-50 to efficiently learn visual features (\({h}_{i}\)) for each spot (\({v}_{i}\)) by maximizing agreement between differently augmented views of the same spot image (\({i}_{i}\)) via a contrastive loss in the latent space (\({l}_{i}\)), and then constructs HSG by the learned visual features\({h}_{i}\).cstMVC model adopting SGATE model learns view-specific representations (\({{p}_{i}}^{1}\)and\({{p}_{i}}^{2}\)) for each of two graphs including HSG and SLG, as well as the latent feature from gene expression data by the autoencoder-based framework as a feature matrix, where a SGATE for each view is trained under weak supervision of the region segmentation to capture its efficient low-dimensional manifold structure, and simultaneously integrates two-view graphs for robust representations (\({r}_{i}\)) by learning weights of different views via attention mechanism.dRobust representations\(R\)can be used for elucidating tumor heterogeneity: detecting spatial domains, visualizing the relationship distance between different domains, and further denoising data. g Total survival rate of patients with the high ( \( > \) median value) or low (low \( < \) median value) expression level of 11 signature genes for domains 10 and 11 in gene expression data of ovarian cancer from TCGA by GEPIA2 [86] (Supplementary Table 1 ). h Immunofluorescent staining of the tissue section and 15 manually segmented tumor regions, where those regions are outlined by their histological annotations: invasive carcinoma (red), carcinoma in situ (yellow), and benign hyperplasia (green). The intensity of DAPI, fiducial frame, and anti-CD3 is shown in green, blue, and yellow. i Spatial clustering by DR-SC, Squidpy, stLearn, BayesSpace, STAGATE, and stMVC. j UMAP visualization of latent features by stMVC. Domains are outlined by their histological annotations. k Heatmap of gene expression of signature genes from five domains enriched in the carcinoma in situ region by stMVC. Rows and columns indicate genes and domains. l Spatial expression of classical marker genes for stromal and immune cells, including PTPRC , CD14 , IGCL2 , IGHG3 , MS4A1 , MYLK , HLA - DRB1 , CD4 , CD8A , ENG , FABP4 , and FCGR3B for data denoised by stMVC. Source data are provided as a Source Data file. Full size image We found that stMVC facilitates detecting more domains enriched for the cancer regions, compared to those by all other computational methods (Fig. 3b–d, i–k and Supplementary Figs. 6b , c, 7 , 8b , c and 9 ). Particularly for the regions outlined with black color on the ovarian cancer, we noted that stMVC detects four domains while other methods detect one or two domains, and also for the regions marked in black on the breast cancer, stMVC detects five regions while other methods detect at most three regions. Additionally, the feature embeddings extracted by stMVC are better separated between those different domains than those by Squidpy, Giotto, DR-SC, stLearn, and STAGATE, and each domain has its specific signature genes named SVGs. To further support the accuracy of detecting cell-states missed by other methods, e.g., four domains of ovarian cancer, we adopted three independent ways. Specifically, we found that (i) the domains 11 and 12 cells are enriched in different cell populations that are not clearly separated in the scRNA-seq data of 4081 epithelial cells of one additional ovarian cancer sample from previous research [30] , by evaluating whether or not the average expression levels of the signature genes between two domains are different or not correlated (Fisher’s exact test, \(p=0.2377\) , Fig. 3e , see Supplementary Methods ), indicating that these cells exist in ovarian cancer, as well as the advantage of SRT data over scRNA-seq data in terms of visualization of the gene expression levels in the context of tissue; (ii) four domains have different functions, which may be influenced by the infiltrating stromal and immune cells (Fig. 3f and Supplementary Fig. 10a, b , Estimation of cell populations for each spot by SpatialDecon [31] in Supplementary Methods ), i.e., domain 10 cells are involved in TNF- \(\alpha\) by infiltrating immune cells such as CD8 + T cell [32] to elevate NF-kB activity for increasing the risk of cancer, and modulating IL-6/STAT3 signaling to create a positive feedback loop for cell proliferation and cancer initiation; [33] domain 11 cells are related to HIF-1 signaling pathway induced by infiltrating cancer-associated fibroblasts (CAFs) [34] , and NRF2 pathway for tumor adaptation to microenvironmental hypoxia [35] ; domain 12 cells show overexpression of matrix metalloproteinases genes [36] , and TGF-beta secreted by infiltrating macrophages [37] , for promoting ovarian cancer metastasis and migration; and domain 13 cells are mediated by VEGFA/VEGFR2 signaling pathway serving a vital function in the angiogenesis of ovarian cancer; [38] and (iii) the expression of signature genes of domains 10 ( \(p=0.036\) ) and 11 ( \(p=0.032\) ) with more enriched CAFs is significantly correlated with shorter overall survival, which was evaluated by an independent ovarian cancer dataset from the TCGA database (Fig. 3g and signature genes in Supplementary Table 1 ). The conclusion is consistent with the previous research that the proportion of CAF in ovarian cancer is associated with a poor prognosis [39] . In addition, we noted that domain 13 cells exhibit over-expression of NEDD9 which is associated with the progression of and an unfavorable prognosis in ovarian cancer [40] . In addition to infiltrating stromal and immune cells, we found that distinct cell-states are surrounded by different microenvironments. For example, among the five domains in the region of carcinoma in situ of breast cancer (Fig. 3i–l and Supplementary Fig. 8d, e ), we noted that domains 13 and 14 are surrounded by more immune cells such as macrophage ( CD14 ), dendritic cell ( HLA-DRB1 ), and T cell ( CD4 and CD8A ); domains 11, 15, and 16 are mostly surrounded by plasma B cell ( IGCL2 and IGHG3 ) and two types of endothelial cell ( FABP4 for endothelial cell_DCN, VWF and ENG for endothelial cell_VWF) defined by our previous study; [41] and domain 15 cells are also surrounded by myofibroblast ( MYLK ) and follicular B cell ( MS4A1 ). Another interesting feature of stMVC is able to distinguish normal cells and cancer cells, by utilizing the histological features where normal cells and cancer cells have different texture features in terms of size and shape. To clarify this, we designed a tumor suppressor gene- and oncogene-based statistical model to detect normal cells (see “Statistical model for detecting normal cells”). For example, in ovarian cancer, we observed that normal cells with over-expression of suppressor genes (i.e., TP53 and BRCA2 ) [42] and lower-expression of oncogenes (i.e., MYC and NME1 ) [43] are mainly enriched in domains 4, 5, 8, and 9, and normal and cancer cells are separated at the UMAP space (Supplementary Fig. 10c–e ). In short, stMVC is more conductive to clarify tissue heterogeneity in terms of detecting normal cells and tumor cells related to cell proliferation and migration in different spatial regions, which has the potential for clinical and prognostic applications. stMVC enables us to identify transited cell-states To further demonstrate the application power of stMVC, we analyzed the result of breast cancer by stMVC to elucidate its intratumoral heterogeneity and infer possible trajectories in cancer development. The elevated expression of human epidermal growth factor receptor (HER)2 and estrogen receptor (ER) throughout the tumor regions and minimal expression of progesterone receptor (PR) for the data from stMVC, which is in line with the clinical report of Luminal B (Supplementary Fig. 11 ). More interestingly, we observed that stMVC (i) detects four domains in the ER + invasive carcinoma region outlined with red color, and the detected domains 10 and 3 are very different from DR-SC, Squidpy, stLearn, BayesSpace, and Giotto; (ii) predicts a possible trajectory between three domains, i.e., domain 6 → domain 10 → domain 3, where the trajectory is also detected by DR-SC, Squidpy and stLearn, and the inferred trajectories by those four computational methods can be further validated by trajectory algorithm PAGA [44] ; and (iii) similar to stMVC, STAGATE can detect domain 10 cells, however, the trajectory detected by it is very distinct from that by other methods, i.e., there is no direct trajectory between domains 10 and 3 (Figs. 3 i and 4a and Supplementary Figs. 8 b and 12a ). Fig. 4: stMVC is able to identify tumor-related cell-states and their transition cell-states from the invasive carcinoma region in the breast cancer sample. a UMAP visualization and PAGA graph generated by the low-dimensional features by stMVC, Squidpy, stLearn, DR-SC, and STAGATE, respectively. The predicted clusters for each method are the same as in Fig. 3i . b Gene expression levels of nine marker genes for three different cell-states on the PAGA graph by the low-dimensional features of stMVC. c Visualization of the clustering and trajectory inference from 2352 epithelial cells of CID4067 (an independent luminal B patient), and pseudo-time-dependent changes in expression levels of KCNK6 , PDZK1IP1 , KGK1 , and ARMT1 . Each color indicates one cluster. d Total survival rate of patients with the high or low expression level of three representative signature genes of domain 10 (i.e., TOP2A , NUAK1 , and PGK1 , \(p=0.022\) ) and domain 3 (i.e., ARMT1 , RMND1 , and TTLL12 , \(p=0.05\) ) in the RNA-seq data of breast cancer from TCGA database. The logrank test was used for the survival analysis. These breast cancer patients were classified into two groups based on their expression (high \( > 30\%\) value, low \( < 70\%\) value) for comparison of survival. Note that 794 samples with Luminal A, Luminal B, and Her2 subtypes by PAM50 were used in our survival analysis. Source data are provided as a Source Data file. Full size image We validated our predictions by the following several independent ways. Specifically, we noted that (i) four domains have different functions, i.e., domain 6 cells show the high expression levels of genes such as LUCAT1 and PDZK1IP1 for regulating breast cancer cell stemness [45] , [46] ; domain 10 cells show overexpression of NUAK1 and TOP2A correlated with the differentiation and stage or grade of the carcinoma [47] , [48] ; domain 3 cells expressing ARMT1 and RMND1 within breast cancer susceptibility locus affect cell proliferation [49] ; and domain 5 cells with overexpression of MMP1 and MMP11 mediate cell invasion and apoptotic process [50] (Fig. 4b and Supplementary Figs. 12 a and 13 ); (ii) by re-analyzing an independent scRNA-seq data of 24,489 epithelial cells from 20 breast cancer samples, the higher expression of ARMT1 and RMND1 is in scRNA-seq data from ER + patients, compared with those from ER − patients (Supplementary Fig. 12b ), which is consistent with the previous conclusion: ER, ARMT1 , and RMND1 are co-expressed [51] , as well as domains 10 and 3 cells existing in breast cancer; (iii) there is a trajectory between three clusters identified from independent scRNA-seq data of 2352 epithelial cells of CID4067 (a representative luminal B patient, Supplementary Fig. 12b ) by Monocle 2 [52] , and with the estimated pseudo-time, the expression of KCNK6 and PDZK1IP1 for domain 6 decreases, ARMT1 for domains 10 and 3 increases, and especially PGK1 for domain 10 is highly expressed at the middle state, supporting our trajectory inference between domains 6, 10, and 3 (Fig. 4c ); and (iv) the average expression of three representative signature genes for domain 10 (i.e., TOP2A , NUAK1 , and PGK1 , \(p=0.022\) ) and 3 (i.e., ARMT1 , RMND1 , and TTLL12 , \(p=0.05\) ) is significantly correlated with shorter overall survival, which was evaluated by independent breast cancer patients from TCGA database (Fig. 4d ). Hence, these results indicate that there is possible cell development from cancer stem cells to malignant cells. Taken together, stMVC can identify cancer-related cell-states and transited cell-states while supporting clinical and prognostic cancer applications from SRT data. stMVC improves the results for detecting layer-specific inhibitory neurons in mouse brain In addition to cancer data from the Visium platform, we further demonstrated stMVC on the mouse primary visual cortex (V1) 1020-gene dataset from the STARmap platform [3] , to detect cell-states from functionally distinct layers. We downloaded RNA clusters per cell predicted by ClusterMap, annotated seven distinct layers (or regions) from raw fluorescence data based on our segmentation strategy (Fig. 5a, b ), randomly selected 70% of manual regions to supervise the training of the stMVC, and visualized 10-dimensional features from stMVC by mapping them into two-dimensional UMAP. Subsequently, for each of the seven layers, we predicted cell clusters by the Louvain algorithm to identify excitatory and inhibitory neurons by checking the distribution of their classical marker genes [53] (Supplementary Fig. 14 ). For comparison, we also applied ClusterMap for spatial clustering and visualization. Fig. 5: stMVC enables the identification of layer-specific excitatory and inhibitory neurons in the mouse primary visual cortex (V1) dataset. a Raw DAPI image of the V1 tissue annotated with seven functionally distinct layers (up panel). Seven representative cells from different layers (bottom panel). b Tissue region map predicted by stMVC and ClusterMap. c UMAP visualization of the latent features by stMVC and ClusterMap. The layer annotation and color for each cell are the same with ( b ). d UMAP visualization (by stMVC) of the marker genes Slc17a7 and Gad1 for excitatory and inhibitory neurons, respectively. e The spatial map of excitatory and inhibitory neurons predicted by stMVC and ClusterMap, respectively. Each color indicates one cluster. f Heatmap of the average gene expression of signature genes for four domains of excitatory neurons in L2-6 by stMVC. Rows and columns indicate genes and different layers, respectively. g Dot plot showing the expression levels of marker genes for different subtypes of inhibitory neurons in L2-6 by stMVC. Source data are provided as a Source Data file. Full size image We found that (i) each cortex layer is assigned almost by different feature embeddings from stMVC, compared to ClusterMap, and the excitatory ( Slc17a7 ) and inhibitory ( Gad1 ) neurons are distributed in the L2/3, L4, L5, and L6 canonical layers (Fig. 5c, d ); (ii) stMVC and ClusterMap can accurately detect the layer-specific distribution of excitatory neurons in the L2-6 layers, i.e., layer-specific genes such as Nov , Rorb , Cplx1 , and Pcp4 are highly expressed in L2/3, L4, L5, and L6, respectively [3] (Fig. 5e, f ). However, stMVC is also able to detect a layer-specific pattern of inhibitory neurons, i.e., Sst + and Pvalb + neurons tend to be enriched in L5-6 layers while Vip + neuron tends to be enriched in L2-4 layers (Fig. 5e, g ), which is consistent with the previous study [53] . The application of the brain dataset further illustrated that stMVC is able to find cell-states related to the distinct functional regions. In this work, we proposed stMVC for analyzing SRT data to disentangle the heterogeneity of tissue, especially for the tumor, which integrates four-layer profiles: histological image data, spatial location, gene expression, and region segmentation (i.e., global position) indicating biological contexts, by attention-based multi-view graph collaborative learning. Such tumor position information in the tissue structure used by stMVC can help us to elucidate intratumoral heterogeneity. Different from previous methods that integrate histology and spatial location data by a user-defined weight, for example, SpaGCN manually adjusts the weight of histology in gene expression smoothing, stMVC adopts an attention-based strategy to automatically learn weights of different views for robust representations. Besides, our feature extraction framework from the ResNet-50 model trained for histological image data by data augmentations and contrastive learning did help stMVC to learn more efficient visual features, compared with those from the pre-trained ResNet-50 mode by ImageNet, which was used by stLearn (see the comparison results between SGATE-HSG and SGATE-HSG-N detailed at Fig. 2b–e and Supplementary Figs. 1 – 6 and 8 ). The evaluations on two real cancer datasets demonstrated the advantages of stMVC described above, which are able to detect cell-states related to cell stemness, migration, and metastasis distributed in different spatial domains, providing biological insights into tumor heterogeneity. In particular, for the breast cancer dataset, we demonstrated potential clinical and prognostic applications from SRT data, by identifying cancer-related cell-states and also transition cell-states missed by competing methods, which were further validated by clinical data. By comparing stMVC with the three SGATE-based single-view models, we found that stMVC has a better performance in terms of clustering, inference of trajectory, and denoising, which is mainly attributed to the collaborative learning of multi-view graphs. Besides, we observed that SGATE-based spatial-location-graph model performs better than SGATE-based histological-similarity-graph model, however, SGATE-based histological-similarity-graph model is able to capture some rich boundary information as a complementary to SGATE-based spatial-location-graph model. Hence, we believed that the perspective of modeling SRT data by multi-view graphs enables a better understanding of the tissue heterogeneity, compared with that by single-view graph. In addition, by comparing with the mean-based strategy stMVC-M, we noted that stMVC achieves better and comparable performance. Specifically, (i) regarding histology without rich texture information, such as DLPFC and ovarian cancer samples, stMVC-M is more vulnerable to the noise signals from the histological visual features while stMVC is easier to capture the finer structure by automatically learning the weight of each of multiple graphs; (ii) regarding histology with rich tissue anatomical structure, like breast cancer sample, both models have a similar result. Hence, we also implemented the mean-based strategy in stMVC model as an option for users to select. As of now, developing models for integrating SRT data from multiple samples are facing several challenges, for example, the batch effect of gene expression data from multiple sources, as well as their sparsity and noise; constructing the association between spots from different physical metric spaces; and removing the artifacts of histology while creating the relationship between multiple samples [54] , [55] . However, we believed that (i) the visual feature extraction model by data augmentations and contrastive learning provides a solution to construct the association of spots between different samples; and (ii) the multi-view graph collaborative learning model can provide a novel perspective to integrate multiple SRT datasets by combining multi-layer profiles data. Besides, stMVC is easily scalable to process spatially resolved chromatin accessibility (ATAC-seq) or proteomics data [56] , [57] , by replacing the feature matrix from gene expression data with that from ATAC-seq or proteomics data. Furthermore, with the advance of spatial multi-omics technology [58] , stMVC can be easily adjusted to adapt by either adding more graphs created by different omics data or substituting the feature matrix from single-omics data with that from multi-omics data fusion [59] , [60] . Similar to single-view GAT models such as STAGATE, stMVC can be applied to analyze the SRT data of other sequencing-based technologies such as Slide-seq [61] and Slide-seqV2 [62] . Additionally, by exploiting spatiotemporal information derived from stMVC, we can calculate spatial (dynamic) network biomarkers [63] , [64] , [65] , [66] or metabolic states [67] , [68] for accurately and reliably quantifying biological systems and further predicting their complex dynamics/behaviors. We benchmarked the running time of stMVC on the simulated datasets by subsampling spots from the human DLPFC datasets. We observed that stMVC is fast, and takes 38 min to process the SRT dataset with 20 K spots. In particular, the running time is approximately linearly related to the number of input spots (Supplementary Fig. 15 ), which is considered as an advantage of stMVC for processing a bigger dataset. In our future work, we will further improve the scalability of stMVC, e.g., by introducing a subgraph sampling training strategy. Some limitations still are found in stMVC: (i) compared with the visual features extraction framework from the ResNet-50 model pre-trained by the ImageNet, the preprocessed step for training SimCLR needs more computational resources and times; and (ii) region segmentation for tumor position is manually annotated based on the staining density of antibodies. With the exploration of deep learning frameworks of generalizable segmentation tools [69] , [70] , we will further investigate creating a more efficient stMVC model with a more automatic architecture in the future study. stMVC model stMVC is a multi-view graph collaborative learning model, which integrates four-layer profiles: gene expression ( \(X\in {R}^{m\times n}\) ), spatial location ( \(S=\left({s}_{1},\ldots,{s}_{n}\right)\in {R}^{n\times 2},{s}_{i}=({s}_{{ix}},{s}_{{iy}})\) ), histological image data ( \(I=\left({i}_{1},\ldots,{i}_{n}\right)\) ), and manual region segmentation ( \(Y={({y}_{1},\ldots,{y}_{n})}^{T}\in {R}^{n\times 1},{y}_{i}\in \{1,\ldots,K\}\) ), where \(m\) , \(n\) , and \(K\) are the number of genes, spots, and spatial domains (manual segmentation), to elucidate tumor heterogeneity (Fig. 1a–d ). Specifically, we (1) learned visual features ( \({h}_{i}\in {R}^{2048\times 1}\) ) for each spot (or cell) image ( \({i}_{i}\) ) by feature extraction network of the ResNet-50 model that was trained by SimCLR framework [71] , and then constructed HSG based on the similarity of the learned visual features ( \({h}_{i}\) ) (Fig. 1b ); (2) separately learned view-specific representations ( \({P}^{m}=\big({{p}_{1}}^{m}\) ,…, \({{p}_{n}}^{m}\big)\in {R}^{d\times n}\) , where \(d\) is the number of latent features, \(m\in \left\{{{{{\mathrm{1,2}}}}}\right\}\) indicating \(m\) th graph) by SGATE for each of two-view graphs: HSG and SLG, as well as low-dimensional feature of \(X\) by an autoencoder as a feature matrix ( \(Z\in {R}^{b\times n}\) , where the default value of \(b\) is 50, indicating the dimension of latent features), and meanwhile automatically learned the weights of two graphs for robust representations ( \(R=({r}_{1},..,{r}_{n})\in {R}^{d\times n}\) ) by attention mechanism, in a semi-supervision manner from region segmentation (Fig. 1c ). Learning visual features by contrastive learning to construct HSG To remove the noise from histology staining and extract morphological information from histological image data, we adopted SimCLR model to efficiently learn visual features for each spot by maximizing agreement between differently augmented views of the same spot image via a contrastive loss in the latent space (Fig. 1b ). For a spot \({v}_{i}\) from the Visium platform, the physical location of which in the tissue slice is represented by \(({s}_{{ix}},{s}_{{iy}})\) , a square containing \(40\times 40\) pixels centered on \(({s}_{{ix}},{s}_{{iy}})\) is regarded as its image \({i}_{i}\) ; and for a cell \({v}_{i}\) from the STARmap platform, a minimum enclosing bounding rectangle for a cell determined by its RNA locations is treated as its image \({i}_{i}\) . The specific model is described as follows: (1) For each image \({i}_{i}\) , we applied a stochastic data augmentation module to randomly transform it into two correlated views for the same image \({i}_{i}\) , denoted as \({{i}_{m}}^{{\prime} }\) and \({{i}_{n}}^{{\prime} }\) , and considered these two views as a positive pair. In this work, we sequentially apply two simple augmentations: random cropping followed by resizing back to the original size; and random color distortions including randomly changing the brightness, contrast, saturation, and hue of an image [71] . (2) We adopted the ResNet-50 framework [24] as a base encoder \(f(\bullet )\) to extract features ( \({h}_{m}\) and \({h}_{n}\) ) from two augmented views ( \({{i}_{m}}^{{\prime} }\) and \({{i}_{n}}^{{\prime} }\) ), where \({h}_{m},{h}_{n}\in {R}^{2048\times 1}\) is the output after average pooling layer. (3) We used a Multilayer Perceptron (MLP) with one hidden layer to obtain latent features \({l}_{m}=g\left({h}_{m}\right)={W}^{\left(2\right)}\sigma \left({W}^{\left(1\right)}{h}_{m}\right)\) where \(\sigma\) is a ‘relu’ function, the first and second layers are set as 512 and 128, respectively, and \({l}_{m}\) is used to define contrastive loss. (4) Given a set \(\left\{{{i}_{k}}^{{\prime} }\right\}\) including a positive pair of examples \({{i}_{m}}^{{\prime} }\) and \({{i}_{n}}^{{\prime} }\) , the contrastive prediction task aims to identify \({{i}_{n}}^{{\prime} }\) in \({\left\{{{i}_{k}}^{{\prime} }\right\}}_{k\ne m}\) for a given \({{i}_{m}}^{{\prime} }\) . The loss function for a positive pair of samples \(({{i}_{m}}^{{\prime} },{{i}_{n}}^{{\prime} })\) is defined as: 
    l_i,j=- logexp (sim(l_m,l_n)/τ )/∑_k=1^2N𝕀_[k m]exp (sim(l_m,l_n)/τ )
 (1) where \({{{\mbox{sim}}}}\left({l}_{m},{l}_{n}\right)=\frac{{{l}_{m}}^{{{{\rm T}}}}{l}_{n}}{||{l}_{m}||{||}{l}_{n}{||}}\) , \({{\mathbb{I}}}_{\left[k\ne m\right]}\in \{{{{{\mathrm{0,1}}}}}\}\) is an indicator function evaluating to 1 if \(k\ne m\) , \(\tau\) denotes a temperature parameter, and \(N\) indicates batch size. For each SRT data, we randomly selected 85% of the spots as the training sets to train the SimCLR model, and the remaining 15% of the spots as the testing set to test it. Adam optimizer with both a \({1e}^{-6}\) weight decay and a \({1e}^{-4}\) learning rate is used to minimize the above loss function. We trained the SimCLR model until 500 iterations, and then calculated the histological similarity between any two spots by calculating the Cosine similarity between learned features \({h}_{u}\) and \({h}_{v}\) from spots \(u\) and \(v\) as follows: \({\cos }\left({h}_{u},{h}_{v}\right)=\frac{{h}_{u}\bullet {h}_{v}}{\left|\left|{h}_{u}\right|\right|{||}{h}_{v}{||}}\) . A Six-nearest neighbor graph for each spot is kept for constructing the HSG \({G}^{1}=(V,{E}^{1})\) , where each vertex \(v\in V\) indicates a spot, and every two vertices in \(V\) are connected by an edge \(e\in {E}^{1}\) . As a comparison, we used the same strategy to construct naïve HSG \({{G}^{1}}^{{\prime} }=(V,{{E}^{1}}^{{\prime} })\) by the feature extracted by feature extraction framework of ResNet-50 pre-trained by ImageNet to validate the effectiveness of our trained visual feature extraction model. Learning robust representations by multiple view graph collaborative learning We used SGATEs for learning view-specific representations in stMVC, where a SGATE for each view was trained under weak supervision of the region segmentation to capture its efficient low-dimensional manifold structure by integrating gene expression with either HSG ( \({G}^{1}\) ) or SLG, ( \({G}^{2}=(V,{E}^{2})\) ) which is constructed by a six-nearest neighbor graph for each spot based on the Euclidean distance of their physical location in the tissue slice [72] , and meanwhile collaboratively integrated them to learn robust representations for each spot (Fig. 1c ). In this work, two graphs ( \({G}^{1}\) and \({G}^{2}\) ) have the same vertex (spot) set but different edges. stMVC for learning view-specific representations For each view graph, a SGATE model aims to learn accurate low-dimensional features with the following inputs: an adjacency matrix ( \({A}^{m}\in {R}^{n\times n}\) ) representing \(m\) th graph \({G}^{m}\) , where \(m\in \left\{{{{{\mathrm{1,2}}}}}\right\}\) , cell labels indicated by region segmentation ( \(Y\) ), and feature matrix \(Z\) learned from gene expression ( \(X\) ) by autoencoder-based framework (see Supplementary Methods ). A GAT can be built by stacking multiple multi-head graph attention layers [73] . Specifically, each layer is defined as: 
    h_i^(l+1)=σ(1/Q∑_q=1^Q∑_j∈N_iα_ij^qW^qh_j^l)
 (2) 
    α_ij^q=exp (LeakyReLU((a^q)^T[W^qh_i^l||W^qh_j^l]))/∑_o∈N_iexp (LeakyReLU((a^q)^T[W^qh_i^l||W^qh_o^l]))
 (3) where \(Q\) indicates the number of head attention and the default value is two, \({{\alpha }_{{ij}}}^{q}\) is normalized attention coefficients computed by the \(q\) th attention mechanism ( \({a}^{q}\) ), \({W}^{q}\) is the corresponding input linear transformation’s weight matrix, \({N}_{i}\) is the neighborhood of spot ( \({v}_{i}\) ) in the graph, \({{h}_{j}}^{l}\) is the input feature of node \(j\) of the \(l\) th layer, and \(\parallel\) is the concatenation operation. The encoder of each GATE model is composed of two layers of GAT, the output dimensions of the first and second layers are set at 25 and 10, 36 and 18, and 32 and 16, for human DLPFC, ovarian, and breast cancer datasets, respectively. The graph embedding for each graph is represented by \({P}^{m}\) . The decoder of each GATE model is defined as an inner product between the embedding: 
    A^m^'=sigmoid(P^mP^mT)
 (4) where \({{A}^{m}}^{{\prime} }\) is the reconstructed adjacency matrix of \({A}^{m}\) . The goal of learning each GATE model is to minimize the cross-entropy between the input adjacency matrix \({A}^{m}\) and \({{A}^{m}}^{{\prime} }\) : 
    L_reconm=-1/n× n∑_i=1^n∑_j=1^n(a_ij^m× log (a_ij^m')+(1-a_ij^m)× log (1-a_ij^m'))
 (5) where \({{a}_{{ij}}}^{m}\) and \({{{a}_{{ij}}}^{m}}^{{\prime} }\) are the elements of the adjacency matrix \({A}^{m}\) and \({{A}^{m}}^{{\prime} }\) in the \(i\) th row and the \(j\) th column of \(m\) th graph, respectively. To capture biological contexts in the tissue, we further extended the use of the GATE model to do spot class prediction \({{Y}^{m}}^{{\prime} }={{{\mbox{softmax}}}}({{W}_{m}}^{(1)}{P}^{m})\) in a semi-supervision manner from region segmentation, and the loss function of which is summarized as follows: 
    L_prem=1/S∑_l=1^S(-∑_i=1^Ky_i log (y_i^m'))
 (6) where \(S\) is the number of labeled spots, \(K\) is the number of classes, and \({y}_{i}\) and \({{{y}_{i}}^{m}}^{{\prime} }\) are the label vector of spot \({v}_{i}\) from the region segmentation and the prediction of the \(m{{{{{\rm{th}}}}}}\) graph, respectively. Taken together, the loss function of each SGATE model is summarized as: 
    L_SGATEm=L_reconm+β L_prem
 (7) where \(\beta\) is a parameter used to control the weight of two loss functions, and the default value is eight. stMVC for multi-view graph collaborative learning After learning view-specific representations \({{p}_{i}}^{m}\) for a spot ( \({v}_{i}\) ) by the \(m\) th SGATE model, we applied the collaborative learning model to integrate different view graphs for its robust representations ( \({r}_{i}\) ). The contribution of each view to \({r}_{i}\) is unavailable, hence, we proposed the attention-based strategy to learn the weight of each graph for the final representations by the following function: 
    r_i=∑_m=1^Mγ_i^mp_i^m
 (8) where \(M\) is the number of views. Inspired by attention-based models emphasizing on capturing more critical information to the current task from abundant information [22] , [74] , we defined the weight of one view for node \({v}_{i}\) using the following function: 
    γ_i^m=exp (a_m·p_i^C)/∑_o=1^Mexp (a_o·p_i^C)
 (9) where \({{p}_{i}}^{C}\in {R}^{2d\times 1}\) is the concatenation of all view-specific representations of spot \({v}_{i}\) , and \({a}_{m}\in {R}^{2d\times 1}\) is feature vector of the \(m\) th view, describing what kinds of spots will consider the \(m\) th view as informative. If \({{p}_{i}}^{C}\) and \({a}_{m}\) have a large dot product, meaning spot \({v}_{i}\) believes that the \(m\) th view is an informative view, and vice versa. To collaboratively integrate different views into the same semantic space [60] , we further leveraged robust representations to fine-tune the learning of each view graph by transferring knowledge from robust representations to each view-specific representations, as well as optimizing the parameters of \({\left\{{a}_{m}\right\}}_{m=1}^{M}\) in semi-supervised manner through a MLP with one hidden layer to do spot class prediction \({{Y}^{{CL}}}^{{\prime} }={{{\mbox{softmax}}}}({W}^{\left(2\right)}\sigma ({W}^{\left(1\right)}R))\) . The corresponding loss functions are defined as follows: 
    L_transfer=∑_i=1^n∑_m=1^Mγ_i^m(r_i-p_i^m)^2
 (10) 
    L_preCL=1/S∑_l=1^S(-∑_i=1^Ky_i log (y_i^CL'))
 (11) In summary, the total loss function for robust representations by collaboratively integrating multiple views is summarized as follows: 
    L_MVC=∑_m=1^ML_reconm+β^'∑_m=1^ML_prem+δL_transfer+φL_preCL
 (12) where \({\beta }^{{\prime} }\) , \(\delta\) and \(\varphi\) are used to control the weights of these regularization terms, and the default values of them are 10, 0.0005, and 100, respectively. Overall, the objective function of our stMVC model can be effectively optimized with the following iterations, specifically, for each iteration, we (i) optimized the parameters of each SGATE model to learn the view-specific representations based on Eq. ( 7 ), as well as Eq. ( 10 ) when the robust representations ( \(R\) ) has been inferred by the Eq. ( 8 ), and followed by inferring \(R\) via Eq. ( 8 ); and (ii) optimized the parameters of all SGATE models and the parameter vectors of all graphs based on Eq. ( 12 ), and then inferred \(R\) based on the optimized stMVC model. We trained the stMVC model until convergence, and then applied \(R\) for the spatial clustering, visualization, and denoising (Fig. 1d ). Datasets and preprocessing SRT data In our study, human DLPFC, ovarian, and breast cancer datasets with paired gene expression and histology were publicly available from the 10X Genomics website. Specifically, (i) DLPFC dataset with 12 slices each is manually annotated with the six cortical layers and WM by the previous study, where the number of spots ranging from 3460 to 4789 with a median of 3844 [26] . Besides, for each slice, we randomly selected manual annotation with the proportion ranging from 0.1 to 0.9 by 0.1, thus generating nine manual annotation sets, which were used to check if or not stMVC can capture the inner structure of tissue by few labels; (ii) ovarian cancer sample with matching gene expression (3493 spots) and immunofluorescence staining with an anti-human CD45 antibody and DAPI; and (iii) breast cancer sample with paired gene expression data (4727 spots) and immunofluorescence staining with an anti-human CD3 antibody and DAPI. In addition, a mouse primary visual cortex (V1) 1020-gene sample with matching gene expression (1365 cells predicted by ClusterMap) and raw immunofluorescence staining with DAPI was available from STARmap platform [3] . scRNA-seq and bulk RNA-seq data To validate our predictions for the sample of ovarian cancer, we extracted 4081 epithelial cells from one ovarian cancer patient from a previous study [30] . Besides, 24,489 epithelial cells were retrieved from 20 breast cancer patients from previous research, including five luminal B, three Luminal A, three HER2 + , seven triple-negative breast cancers (TNBCs), one HER2 + and ER + , and one normal [75] , to support our findings, and the subtypes are determined by their clinical reports and predictions. Furthermore, the bulk RNA-seq and clinical data of breast cancer in TCGA database were downloaded from the Xena platform for survival analysis [76] , and the PAM50 subtype classifications of breast cancer of TCGA were downloaded from previous research [77] . Preprocessing The top 2000 highly variable genes by the ‘vst’ method of Seurat [78] for each gene expression data from the Visium platform, and all 1020 genes of the mouse primary visual cortex dataset from the STARmap platform, were used to comprehensively compare each computational method. Besides, to efficiently capture the information within gene expression data, we mapped each data into 50-dimensional latent features based on our designed autoencoder-based framework (see Supplementary Methods ), and took them as the input of stMVC. Manual region segmentation We designed a strategy to define biological contexts in each tumor tissue based on the following assumptions: (1) the colors of the antibodies on the immunofluorescence staining of the tumor histology can roughly define the tumor region; (2) cells belonging to the same cell type but are separated by other cells such as immune or other mesenchymal cells may have different cell-states; and (3) the majority of cells in the tumor region are tumors while a few are normal epithelial and infiltrating stromal or immune cells, and the tumor purity was larger than 70%, which was estimated by over 9300 tumors of 21 cancer types from the TCGA database [79] (Supplementary Fig. 16 ). After annotating different regions in the histology image by labelme software [80] , we further applied the OpenCV package [81] to determine the region (or context) to which each spot ( \({v}_{i}\) ) belongs, by calculating the proportion between area of the intersection between a square ( \({{{\mbox{IR}}}}_{i}\) ) containing \(40\times 40\) pixels centered on \(({s}_{{ix}},{s}_{{iy}})\) and a region ( \({R}_{j}\) ), compared to the square. The function is defined as follows: 
    Proportion=Intersection(IR_i,R_j)/IR_i
 (13) By setting \({{\mbox{Proportion}}}\ge 0.5\) , for the ovarian cancer sample, 1658 spots were separately classified into 17 different regions in the tumor, and the remaining 1835 spots in the non-tumor region were treated as the 18th region (Supplementary Fig. 6a ); and for the breast cancer sample, 2091 spots were classified into 15 different regions in the tumor, and the remaining 2636 spots were regarded as the 16th region (Supplementary Fig. 8a ). In addition, we further extended the protocol to process imaging-based SRT data. Specifically, we predicted RNA clusters for each cell by ClusterMap; for each cell \({v}_{i}\) , treated a minimum enclosing bounding rectangle containing the cell determined by its RNA’s physical locations as \({{{\mbox{IR}}}}_{i}\) ; and adopted Eq. ( 7 ) to predict the region to which the cell belongs. By computing, for the mouse V1 sample, 1365 cells were classified into seven regions (Fig. 5b ). Evaluation of denoising of gene expression data We adopted a GI-based measure [60] to quantify the quality of denoised gene expression data by estimating a degree of inequality in the distribution of known layer-specific gene expression levels. Specifically, for each domain of the ground truth, the average expression of each marker gene was calculated; and then the GI for each gene calculated by the ‘gini’ function from reldist package was used to evaluate the specific level of the marker gene [82] . The higher the GI score, the better the denoised data. 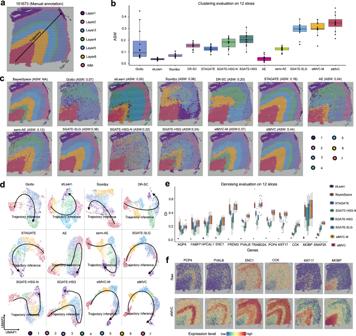Fig. 2: stMVC is able to detect spatial domains, visualize the relationship distance between different domains, and denoise data on the DLPFC dataset. aAnnotation of seven DLPFC layers in slice 151673 by the previous study26, and the spatial adjacency and chronological order between these layers are WM → Layer6 → Layer5 → Layer4 → Layer3 → Layer2 → Layer1.bBoxplot of clustering accuracy in terms of average silhouette width (ASW) for assessing the closeness of multi-view joint features of same cluster compared to the other clusters, on alln= 12 samples. In the boxplot, the center line, box limits and whiskers separately indicate the median, upper and lower quartiles and 1.5 × interquartile range.cSpatial domains detected by BayesSpace, Giotto, stLearn, Squidpy, DR-SC, STAGATE, AE, semi-AE, the three SGATE-based single-view models, stMVC-M, and stMVC on slice 151673.dScatter plot of the two-dimensional UMAP extracted from the latent features by Giotto, stLearn, Squidpy, DR-SC, STAGATE, AE, semi-AE, three SGATE-based single-view models, stMVC-M, and stMVC on slice 151673. Note that the trajectory between seven layers or domains is consistent with (a), and for each method, the predicted clusters and their colors are the same as (c). Note that subplotb–dBayesSpace cannot calculate ASW and visualized using UMAP.eBoxplot of the Gini-index (GI) score of gene expression data denoised by stLearn, BayesSpace, STAGATE, the three SGATE-based single-view models, stMVC-M, and stMVC forn= 12 samples. The higher GI score, the better the denoised data. In the boxplot, the center line, box limits and whiskers indicate the median, upper and lower quartiles and 1.5 × interquartile range, respectively.fSpatial expression of layer-specific genes:26PCP4,PVALB,ENC1,CCK,KRT17, andMOBPfor slice 151673 data denoised by stMVC, where we also provide raw data as a comparison. Source data are provided as a Source Data file. The marker genes used in DLPFC dataset were downloaded from the previous study [26] (Supplementary Table 2 ). Statistical model for detecting normal cells To clarify that stMVC is able to distinguish normal cells from cancer cells by integrating the histological features, we further designed a statistical-based measure to detect normal cells from SRT data. Specifically, we reasoned that (1) normal cells tend to be with a higher expression of tumor suppressor genes while cancer cells tend to have a higher expression of oncogenes; and (2) the expression levels between the tumor suppressor genes and the oncogenes are different or not correlated, which were calculated by Fisher’s exact test (see Supplementary Methods ). Hence, cells with a higher expression of suppressor genes but a lower expression of oncogenes were regarded as the normal cells, noting that the expressions of suppressor genes and the oncogenes are not correlated ( p -value > 0.05). Clustering and visualization After applying stMVC in analyzing SRT data, we learned the accurate low-dimensional representations ( \(R\) ) representing the relationship between any two spots. To further clarify tissue heterogeneity, given \(R\) as the input, we adopted ‘FindNeighbors’ and ‘FindClusters’ function with default parameters from the Seurat package to determine \(k\) -nearest neighbors (KNNs) for each spot, construct the shared nearest neighbor graph, predict the cell clusters by the Louvain algorithm, and each cluster is considered as a spatial domain. We utilized the UMAP algorithm to map the low-dimensional features from each computational method to two-dimension, visualized the distance of cell embeddings between different cell populations by ‘Dimplot’ function, and visualized the clusterings and gene expression patterns at the spatial level by ‘SpatialDimPlot’ and ‘SpatialFeaturePlot’ function, respectively. Evaluation of the clustering We adopted two different metrics to evaluate the clustering by calculating the similarity of features between spots within the predicted cell clusters. Specifically, ROGUE [28] , an entropy-based statistic to quantify the homogeneity of identified cell clusters based on transcriptome similarity between spots within each cluster, and the higher the value, the better the clustering; silhouette width [29] , a measure of how similar a spot is to its predicted cluster compared to other clusters, and the higher the value, the spot well belongs to its cluster, which is calculated as follows: 
    SW(i)=c(i)-d(i)/max {c(i),d(i)}
 (14) where \(d(i)\) , and \(c\left(i\right)\) indicate the average Euclidean distance of the learned low-dimensional joint features between a spot ( \(i\) ) and other spots in the same cluster, and the spot ( \(i\) ) to all spots in the nearest cluster where \(i\) does not belongs, respectively. The average of silhouette width of all spots as the final metrics (ASW) to evaluate clustering performance. 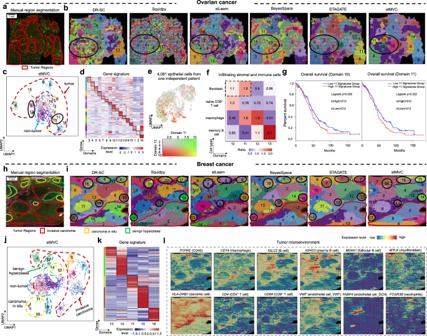Fig. 3: stMVC enables the detection of cell-states distributed in different spatial domains on ovarian and breast cancers. aImmunofluorescent staining of the tissue section and 17 manually segmented tumor regions. The intensity of DAPI, cytokeratin, and CD45 is shown in blue, green, and yellow.bSpatial clustering by DR-SC, Squidpy, stLearn, BayesSpace, STAGATE, and stMVC.cUMAP visualization of latent features by stMVC. Each domain is outlined by the region it belongs to, i.e., tumor or non-tumor.dHeatmap of average gene expression of signature genes from 16 domains by stMVC. Rows and columns indicate genes and domains.eUMAP plot of average expression of signature genes for domains 11 and 12 in scRNA-seq data of 4081 epithelial cells from one independent ovarian cancer.fEnrichment of infiltrating stromal and immune cells in each domain compared to the total distribution of those in four domains. The ratio is calculated by chi-square test85. The larger the ratio, the more cells are enriched in the domain.gTotal survival rate of patients with the high (\( > \)median value) or low (low\( < \)median value) expression level of 11 signature genes for domains 10 and 11 in gene expression data of ovarian cancer from TCGA by GEPIA286(Supplementary Table1).hImmunofluorescent staining of the tissue section and 15 manually segmented tumor regions, where those regions are outlined by their histological annotations: invasive carcinoma (red), carcinoma in situ (yellow), and benign hyperplasia (green). The intensity of DAPI, fiducial frame, and anti-CD3 is shown in green, blue, and yellow.iSpatial clustering by DR-SC, Squidpy, stLearn, BayesSpace, STAGATE, and stMVC.jUMAP visualization of latent features by stMVC. Domains are outlined by their histological annotations.kHeatmap of gene expression of signature genes from five domains enriched in the carcinoma in situ region by stMVC. Rows and columns indicate genes and domains.lSpatial expression of classical marker genes for stromal and immune cells, includingPTPRC,CD14,IGCL2,IGHG3,MS4A1,MYLK,HLA-DRB1,CD4,CD8A,ENG,FABP4, andFCGR3Bfor data denoised by stMVC. Source data are provided as a Source Data file. 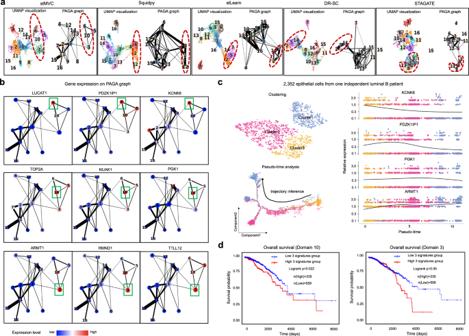Fig. 4: stMVC is able to identify tumor-related cell-states and their transition cell-states from the invasive carcinoma region in the breast cancer sample. aUMAP visualization and PAGA graph generated by the low-dimensional features by stMVC, Squidpy, stLearn, DR-SC, and STAGATE, respectively. The predicted clusters for each method are the same as in Fig.3i.bGene expression levels of nine marker genes for three different cell-states on the PAGA graph by the low-dimensional features of stMVC.cVisualization of the clustering and trajectory inference from 2352 epithelial cells of CID4067 (an independent luminal B patient), and pseudo-time-dependent changes in expression levels ofKCNK6,PDZK1IP1,KGK1, andARMT1. Each color indicates one cluster.dTotal survival rate of patients with the high or low expression level of three representative signature genes of domain 10 (i.e.,TOP2A,NUAK1, andPGK1,\(p=0.022\)) and domain 3 (i.e.,ARMT1,RMND1, andTTLL12,\(p=0.05\)) in the RNA-seq data of breast cancer from TCGA database. The logrank test was used for the survival analysis. These breast cancer patients were classified into two groups based on their expression (high\( > 30\%\)value, low\( < 70\%\)value) for comparison of survival. Note that 794 samples with Luminal A, Luminal B, and Her2 subtypes by PAM50 were used in our survival analysis. Source data are provided as a Source Data file. 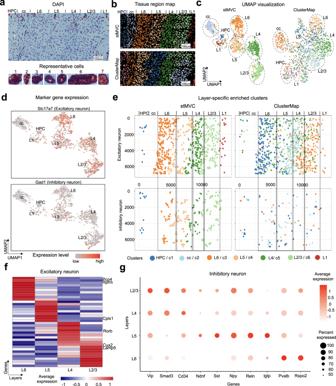Fig. 5: stMVC enables the identification of layer-specific excitatory and inhibitory neurons in the mouse primary visual cortex (V1) dataset. aRaw DAPI image of the V1 tissue annotated with seven functionally distinct layers (up panel). Seven representative cells from different layers (bottom panel).bTissue region map predicted by stMVC and ClusterMap.cUMAP visualization of the latent features by stMVC and ClusterMap. The layer annotation and color for each cell are the same with (b).dUMAP visualization (by stMVC) of the marker genesSlc17a7andGad1for excitatory and inhibitory neurons, respectively.eThe spatial map of excitatory and inhibitory neurons predicted by stMVC and ClusterMap, respectively. Each color indicates one cluster.fHeatmap of the average gene expression of signature genes for four domains of excitatory neurons in L2-6 by stMVC. Rows and columns indicate genes and different layers, respectively.gDot plot showing the expression levels of marker genes for different subtypes of inhibitory neurons in L2-6 by stMVC. Source data are provided as a Source Data file. Identification of SVGs We constructed KNN graph for each spot based on the learned low-dimensional representations ( \(R\) ), and adopted the KNN-smoothing algorithm to aggregate information from 15 nearest spots for each spot to denoise the gene expression data. Then, we identified SVGs from 2000 highly variable genes among different spatial domains from the stMVC model by ‘FindAllMarkers’ from Seurat package. Reporting summary Further information on research design is available in the Nature Research Reporting Summary linked to this article.